Driving diffusionless transformations in colloidal crystals using DNA handshaking Many crystals, such as those of metals, can transform from one symmetry into another having lower free energy via a diffusionless transformation. Here we create binary colloidal crystals consisting of polymer microspheres, pulled together by DNA bridges, that induce specific, reversible attractions between two species of microspheres. Depending on the relative strength of the different interactions, the suspensions spontaneously form either compositionally ordered crystals with CsCl and CuAu-I symmetries, or disordered, solid solution crystals when slowly cooled. Our observations indicate that the CuAu-I crystals form from CsCl parent crystals by a diffusionless transformation, analogous to the Martensitic transformation of iron. Detailed simulations confirm that CuAu-I is not kinetically accessible by direct nucleation from the fluid, but does have a lower free energy than CsCl. The ease with which such structural transformations occur suggests new ways of creating unique metamaterials having structures that may be otherwise kinetically inaccessible. DNA has emerged as a versatile and effective means of directing the self-assembly of microscopic [1] , [2] , [3] and nanoscopic [4] , [5] , [6] , [7] , [8] , [9] particles into a variety of crystalline structures. Such crystals are stabilized by DNA handshaking [10] —the formation of transient DNA bridges between particles bearing complementary DNA sequences—that induces a force drawing the particles together [1] , [11] , [12] , [13] , [14] . Unlike other particle interactions based upon electrostatics or polymers, DNA handshaking permits the engineering of a matrix of specific attractive interactions between a number of particle species—where only species bearing complementary DNA are attracted to one another—and results in particle-based model materials with potentially very rich phase behaviour. Although this approach has yielded a wealth of crystal structures, how these structures nucleate, grow, anneal and whether they can structurally transform like conventional atomic materials remains largely unknown. Here we create suspensions consisting of two species of same-sized, sub-micron spheres that explore a two-dimensional phase diagram parameterized by the strength of the interactions among and between the two species; the interactions themselves being a function of temperature. Specifically, by adjusting the relative amount of different DNA strands on the particle surfaces, we create a sequence of samples that, as the temperature is gradually reduced, fan out over the phase diagram, and that yield crystals whose three-dimensional structure and compositional ordering can be directly visualized using confocal fluorescence microscopy. Depending on their DNA-induced interactions, we find that different samples either yield mixtures of two different types of well-ordered crystals, CsCl and CuAu-I, or randomly substituted, solid-solution crystals having a face-centered-cubic (FCC) structure (FCC-SS). Comparing our findings to simulations of crystal growth [15] and free-energy calculations, based upon a verified model for the DNA interaction [13] , we conclude that the CuAu crystals are formed via a diffusionless transformation [16] from CsCl parent crystals. As often occurs in metal alloys, our crystals spontaneously change from the one that nucleates and grows, into a new lower free-energy crystal structure as the temperature is lowered. This conclusion is made compelling by the observation of several crystallites containing both crystal symmetries joined coherently along a habit plane, as well as other details of the crystallites’ structure. The observed diffusionless transformation results in a net tetragonal deformation analogous to the classical Bain model [17] for the Martensitic transformation of iron from body-centered cubic (BCC) to FCC. More broadly, our findings suggest that many of the complex structural transformations observed in atomic solids, which are exploited to produce specific microstructures through material processing, may have analogues in the behaviour and processing of DNA-linked particle materials. Moreover, our work underscores the utility of existing materials science principles and simulation techniques for understanding these materials and guiding the processes used to form them. Particle interaction design and crystallization We produce suspensions of two mixed particle species, ‘A’ and ‘B’, consisting of same-sized 400 nm diameter polystyrene microspheres, differentiated by their fluorescent tags and the type of DNA sequences grafted [18] uniformly over their surfaces (see Methods for details). Colloidal crystallization is driven by attractive interactions [13] , [14] owing to the formation of DNA bridges between particles bearing complementary DNA strands ( Fig. 1 ). We modulate the three different attractive interaction strengths in the system, E AB , E AA and E BB , by mixing two different DNA strands on each particle surface at a stoichiometric ratio α . Specifically, the A particles contain proportion α of one DNA strand and proportion (1− α ) of its complement, with the proportions reversed on the B particles ( Fig. 1 ). This arrangement naturally leads the ‘unlike’ attractions to be stronger than the ‘like’ attractions ( E AB > E AA , E BB ), avoiding simple phase separation, and the two ‘like’ attractions to be equal ( E AA = E BB ). To form symmetric AB-type alloys, we grew crystals from equimolar mixtures of A and B spheres. Samples with varying ratios of ‘like’ and ‘unlike’ interactions were prepared (by varying the DNA-mixing ratios, 0 ⩽ α ⩽ 0.50), concentrated to ~20% particle volume fraction, sealed in microcentrifuge tubes and submerged in a thermally insulated hot water bath ( T ≈40 °C) (see Methods for details). The passive cooling of this bath, at a rate of ~0.3 °C per h, leads the attractive DNA interaction strength to increase monotonically in time as DNA bridge formation becomes more thermodynamically favourable. Crystal nucleation and growth occur near the DNA duplex melting temperature T m , measured to be in the range 32.5 °C< T m <36.5 °C depending on α . The particle interactions are effectively irreversible once the samples reach room temperature. 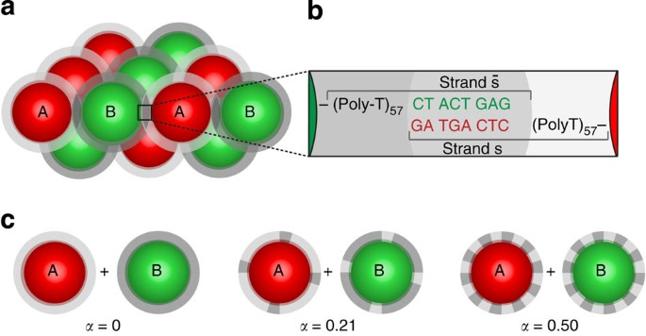Figure 1: Particle bridging by DNA molecules can drive the formation of colloidal crystals. (a) Binary crystals of 400 nm diameter colloids (tagged with different fluorescent dyes) are stabilized by bridges (b) formed between grafted 65-base DNA oligonucleotides containing terminal, complementary 8 base-pair sequences (see Methods). (c) To modulate the relative strength of the resulting interactions between and among the two populations, varying amounts of both strands are attached uniformly to each microsphere, described by a mixing ratioα, as described in the text. Figure 1: Particle bridging by DNA molecules can drive the formation of colloidal crystals. ( a ) Binary crystals of 400 nm diameter colloids (tagged with different fluorescent dyes) are stabilized by bridges ( b ) formed between grafted 65-base DNA oligonucleotides containing terminal, complementary 8 base-pair sequences (see Methods). ( c ) To modulate the relative strength of the resulting interactions between and among the two populations, varying amounts of both strands are attached uniformly to each microsphere, described by a mixing ratio α , as described in the text. Full size image The crystals formed during such slow quenches are diluted and inspected using differential interference contrast and confocal fluorescence microscopy ( Fig. 2 ). In each sample, nearly all of the assemblies display clear crystalline order and faceting ( Supplementary Movies 1 and 2 ) and disordered aggregates contain <5% of the total microparticles. Control experiments at a higher quench rate, ~2 °C per h, and α =0 did not lead to a significant change in crystal morphology or structure. Rapidly quenched experiments on the microscope were observed to form crystals in <1 h, much less than the estimated crystal sedimentation time in our water bath experiments. Experiments at lower volume fractions and selected α values showed little change in crystal morphology at 15% volume fractions, significant reductions in crystallite size and order at 10% volume fractions and no crystals at lower volume fractions. These trends versus volume fraction resemble those for homogeneously nucleated crystals formed using the depletion interaction. Taken together, these findings suggest our crystals form by homogeneous nucleation and growth in a three-dimensional suspension. 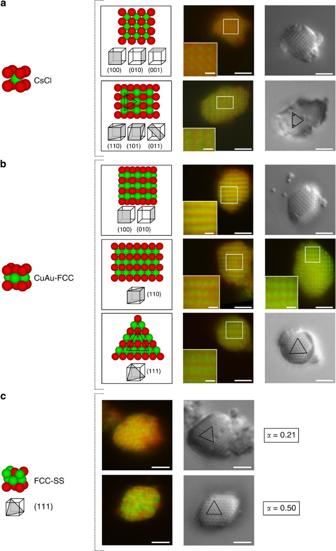Figure 2: Real-space crystallography reveals DNA-directed particle crystals having different structures. Samples prepared with differentαvalues, and thus different interactions, yield crystals having (a) CsCl structure, (b) CuAu-I structure and (c) substitutionally disordered solid-solution FCC (FCC-SS). For each structure, typical facet planes are shown schematically along with corresponding two-colour confocal and DIC (differential interference contrast) micrographs. Scale bars correspond to 2 and 0.5 μm in insets. Figure 2: Real-space crystallography reveals DNA-directed particle crystals having different structures. Samples prepared with different α values, and thus different interactions, yield crystals having ( a ) CsCl structure, ( b ) CuAu-I structure and ( c ) substitutionally disordered solid-solution FCC (FCC-SS). For each structure, typical facet planes are shown schematically along with corresponding two-colour confocal and DIC (differential interference contrast) micrographs. Scale bars correspond to 2 and 0.5 μm in insets. Full size image Optical imaging of colloidal crystals Real-space crystallography of colloidal crystals typically requires refractive index matching to avoid light scattering, but this is impractical in our system owing to the necessity of using water as a solvent for DNA. Instead, we adjusted the particle diameter to a size range (~400 nm) that is small enough to minimize light scattering, rendering the crystals effectively transparent, while still large enough to allow optical imaging above the diffraction limit. Our 400 nm particles are 3–5 times smaller in diameter (or 30–120 times smaller in volume) than those typically used in confocal studies of index-matched colloidal crystals, which does lead to a reduction in both overall colour contrast and signal to noise compared with earlier studies. Confocal imaging of crystallites of large, non-index matched particles can often show apparent three-dimensional periodicity because of the complex process of light scattering and propagation in a periodic dielectric structure. In such cases, the observed brightness maxima do not necessarily correspond to individual particles, but rather anti-nodes of a complex three-dimensional interference pattern. To confirm that our confocal images are not artifactual diffraction patterns, we collected two-colour scans on selected crystallites in the third, z-direction ( Supplementary Movies 3 , 4 , 5 , 6 , 7 , 8 , 9 , 10 , 11 ). Three features of these z-scan data support our conclusion that we are observing crystal structure rather than merely diffraction patterns: (i) careful scrutiny detects point and planar defects deep inside multiple crystallites ( Supplementary Movies 5 , 8 , 9 ); (ii) the appearance of two-colour contrast deep within crystals (as all particles would scatter light similarly, a diffracted/scattered light field would illuminate both particle species equally, Supplementary Movies 3 , 4 , 5 , 6 , 7 , 8 , 9 , 10 , 11 ); and (iii) differential interference contrast in midplanes of the crystals indicates that white light transillumination is not significantly depolarized by passing through the crystallites, as it would be in a strongly scattering sample ( Supplementary Movies 1 , 2 ). The confocal depth of focus (~500 nm), however, is comparable in size to our unit cells, preventing us from resolving individual crystal planes in the vertical direction; three-dimensional fluorescence data do not show clearly resolvable periodicity in the z-direction. Each confocal image is likely the sum of fluorescent intensity in at least two vertically adjacent crystal planes. In all but one case, our crystal structures consist of vertical columns of A and B particles ( Supplementary Fig. S1 ), therefore this blurring in z does not decrease in-plane fluorescence periodicity. In the remaining case, finite z resolution blurs the in-plane fluorescence periodicity only slightly, shown in Supplementary Fig. S2 . Real-space crystallography The crystal structures of a number of crystallites in each sample were determined by obtaining a confocal image in their midplane and matching the two-dimensional periodicity of fluorescence to geometrical models, as summarized in Supplementary Table S1 . The samples with the weakest ‘like’ interactions ( α values <0.10) predominantly showed crystals having a CsCl structure ( Fig. 2a ), samples with intermediate strength ‘like’ interactions yielded a mixture of CsCl and CuAu-I crystals ( Fig. 2b ), and those with the strongest ‘like’ interactions showed solid-solution crystals having an FCC symmetry ( Fig. 2c ). The CsCl and CuAu-I structures are ordered superlattices of BCC and FCC structures, respectively. In both structures, each particle has eight neighbours of the opposite species, while in the CuAu phase each particle additionally has four ‘like’ neighbours. The FCC solid-solution crystals, while structurally ordered, exhibit a large amount of compositional disorder. 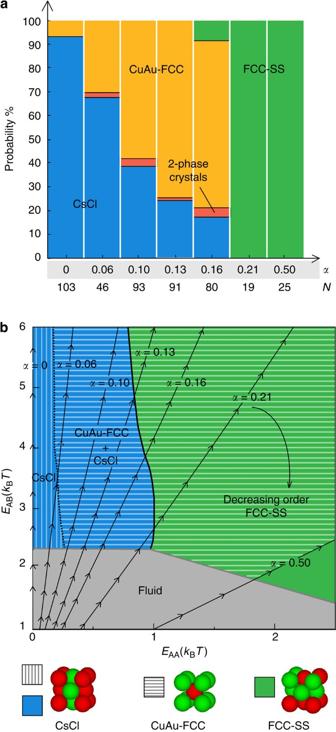Figure 3: Possible crystal structures and computed binary phase diagram arising from mixed DNA-particle architecture. (a) Probabilities of observed crystal structures for experimentally realizedαvalues.Nrepresents the number of crystals whose crystallography was analysed, 457 in total. Detailed statistics are reported inSupplementary Table S2. (b) A phase diagram that displays both the phases that nucleate and grow from the fluid, CsCl (blue) and FCC solid solutions (green), as well as the structures that have the lowest free energy, CsCl (vertical stripes) or CuAu-FCC (horizontal stripes). Computed sample trajectories across the phase diagram, for experimentally realized values ofα, are represented by rays in black, arrowheads at 1 °C intervals. Figure 3a summarizes the frequency of occurrence for these three different structures, as a function of the α -controlled ‘like’ interaction strength. The data show an increasing proportion of CuAu crystals as ‘like’ interactions are increased, followed by an abrupt change to FCC-SS for α >0.16. Previously, CsCl [19] and CuAu [20] colloidal crystals have been observed in much larger, oppositely charged colloids, but not with DNA handshaking interactions. The phase diagrams and transitions between these charged crystal structures were also studied theoretically [20] for interactions relevant to those materials. Figure 3: Possible crystal structures and computed binary phase diagram arising from mixed DNA-particle architecture. ( a ) Probabilities of observed crystal structures for experimentally realized α values. N represents the number of crystals whose crystallography was analysed, 457 in total. Detailed statistics are reported in Supplementary Table S2 . ( b ) A phase diagram that displays both the phases that nucleate and grow from the fluid, CsCl (blue) and FCC solid solutions (green), as well as the structures that have the lowest free energy, CsCl (vertical stripes) or CuAu-FCC (horizontal stripes). Computed sample trajectories across the phase diagram, for experimentally realized values of α , are represented by rays in black, arrowheads at 1 °C intervals. Full size image Free-energy calculations and non-equilibrium simulations The complex outcome of our experiments was illuminated using a comprehensive suite [15] of calculations based on a recently developed coarse-grained interaction potential model for DNA-mediated binding between pairs of spherical colloidal particles [13] . First, free-energy calculations were employed to compare the stability of the competing ideal binary superlattice structures (CuAu-I and CsCl). The calculations were based primarily on the quasi-harmonic approximation (QHA) [21] in which the free energy is assumed to be comprised of vibrational entropic and enthalpic contributions. Within the QHA, the vibrational entropy is computed within a harmonic theory but includes a correction for anharmonic effects by accounting for the thermal expansion predicted by the interaction potential. The QHA predictions were validated using a more computationally expensive approach based on thermodynamic integration [22] . The free-energy calculations were then combined with results of non-equilibrium Monte Carlo (NEMC) simulations [15] . There, binary mixtures of particles, initially in a disordered fluid state, were evolved and allowed to spontaneously form crystallites with varying degrees of compositional defects (for example, antisites). The NEMC results, which provide a link between interaction potential parameters and compositional ordering, were then used to inform additional free-energy calculations, thereby enabling estimation of free energies for kinetically accessible, rather than the ideal, structures. For small values of ‘like’ attraction, NEMC simulations show that CsCl crystallites nucleate homogeneously and grow with essentially perfect ordering (blue shaded region on the left in Fig. 3b ). For large values of ‘like’ attraction (green region on the right), simulations find that the two species co-crystallize into FCC crystals with partial compositional order corresponding to the experimentally observed FCC-SS structure. Although a perfectly ordered, close-packed superlattice could have lower free energy than the FCC-SS structure, it is not kinetically accessible from the fluid phase—weakly attractive sites present on the growing FCC crystal surface bind new particles in the ‘wrong’ locations, frustrating ordered growth [15] . The operational boundary between CsCl and FCC-SS growth in simulation roughly corresponds to the point where the as grown FCC-SS becomes the lower free-energy state despite its disorder [15] . Notably, the free-energy calculations show that the perfect close-packed superlattice has lower free energy than CsCl and FCC-SS over much of the phase diagram (horizontal stripes in Fig. 3b ). The CsCl structure has the lowest free energy only for very small ‘like’ binding, despite its lower-binding energy, by virtue of the higher vibrational entropy of its floppy structure. Computed phase trajectories We use a quantitative model for DNA-induced interactions to model the trajectories taken by our different samples across the phase diagram. Detailed calculations of the three temperature-dependent attractions ( E AB , E AA and E BB ) using a recently published [13] , empirically validated model show them to be roughly proportional across a broad range of temperatures T . As the temperature is slowly reduced, each sample follows a different trajectory across the phase diagram that radiates outward from the origin at an ‘angle’ dictated by α ( Fig. 3b ). Observing CuAu crystals is thermodynamically expected by virtue of their lowest free energy, but we are left with the crucial question of how they form. Hypothetical mechanisms would include: (i) direct nucleation and growth from the fluid; (ii) formation from the FCC-SS structures by annealing; and (iii) a solid–solid transformation from another crystal structure. The first case is wholly incompatible with our simulations, while the second case is unlikely given the absence of solid diffusion in these systems. Neither of the first two hypotheses explain why the CuAu phase abruptly disappears for α >0.16, despite significant thermodynamic driving favouring CuAu over FCC-SS. In what follows we will present evidence that indicates that the CuAu crystals are formed by a diffusionless transformation from CsCl parent crystals. Unlike earlier observations of diffusionless transformations in other colloidal systems, driven by electric fields [23] or confinement [24] , our crystallites transform spontaneously when the temperature is changed. Were the CuAu crystals formed from CsCl parent crystals, it would explain why the two structures are always found in apparent coexistence, or equivalently, why the CuAu phase disappears abruptly above the same α threshold as CsCl, only samples with α <0.16 pass inside the phase domain for which the nucleation and growth of CsCl are thermodynamically favourable relative to FCC-SS ( Fig. 3b ). A diffusionless transformation from a well-ordered parent phase (CsCl) would create a child phase (CuAu) with similarly perfect compositional ordering. Such a diffusionless transformation is physically plausible because of the fact that both crystal structures are connected by a simple tetragonal deformation with extension along a CsCl [100] direction ( Supplementary Fig. S4 ), analogous to the classical Bain description of the Martensitic transformation between BCC and FCC forms of iron [16] , [17] . Moreover, as the lattice dimensions in the two perpendicular directions can contract to maintain constant nearest-neighbour separation, a uniform tetragonal deformation in CsCl has no enthalpic penalty—it is a ‘floppy mode’. The specific microscopic pathway by which the transformation proceeds, however, could not be experimentally observed in situ . Direct experimental evidence for a diffusionless transformation was found in seven ‘two-phase’ crystallites, each containing two distinct domains having CsCl and CuAu structure, divided by a sharp, straight interface showing them joined coherently ( Fig. 4 and Supplementary Movie 11 ). In atomic materials, boundaries between parent and child phases are typically oriented along so-called habit planes dictated by the geometry of the transformation as well as the commensurability of the two lattices and elastic strain minimization. Indeed, each of the seven two-phase crystals we observed displayed precisely the same crystallographic orientation of the two domains relative to each other and the interface between them, as expected for a single preferred habit plane in an isolated crystallite. Specifically, continuous rows of ‘like’ particles between {110} of CsCl and {100} of CuAu form a ~100° angle, which allows for two-dimensional commensurability of the two crystal facets in the focal plane along a common, close-packed chain of alternating A and B particles. Confocal scans indicate that the habit plane continues in the z-direction, with minimal tilt with respect to the focal plane. The precise three-dimensional orientation of the habit plane in these crystals could not be reliably determined by confocal microscopy. Two possible interpretations for the habit plane orientation are that the (011) plane of CsCl is joined to the (111) plane of CuAu or that the (112) plane of CsCl is joined to the (101) plane of CuAu ( Supplementary Fig. S3 ). The former corresponds to the shear plane predicted by the the Kurdjumov–Sachs (KS) and Nishiyama–Wasserman (NW) models [25] of the transformation between α -Fe (BCC) and γ-Fe (FCC) phases. 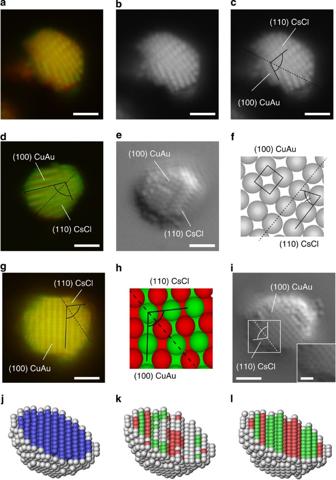Figure 4: Habit plane observations and simulations provide evidence for diffusionless transformations. Multiple crystals—one crystal per row—displayed one or two habit plane interfaces between CsCl and CuAu phases. As shown in confocal micrographs (a–d,g), the domains join coherently at the particle scale, with a consistent 100° angle between (110) of CsCl and (100) of CuAu. Scale bars correspond to 2 μm. A 100° angle allows the (110) and (100) planes of the two phases to join commensurably in the plane of viewing, shown schematically (h). Differential interference contrast (DIC) micrographs (e,i) reveal the corresponding habit plane structure, shown schematically (f). MMC simulations show an initial CsCl crystal (j) transforming (k) into a stable final CuAu-FCC structure with HCP-like stacking faults (l). Images show a rendered section through the crystallite, coloured using common neighbour analysis: blue (BCC), red (HCP) and green (FCC). Figure 4: Habit plane observations and simulations provide evidence for diffusionless transformations. Multiple crystals—one crystal per row—displayed one or two habit plane interfaces between CsCl and CuAu phases. As shown in confocal micrographs ( a – d , g ), the domains join coherently at the particle scale, with a consistent 100° angle between (110) of CsCl and (100) of CuAu. Scale bars correspond to 2 μm. A 100° angle allows the (110) and (100) planes of the two phases to join commensurably in the plane of viewing, shown schematically ( h ). Differential interference contrast (DIC) micrographs ( e , i ) reveal the corresponding habit plane structure, shown schematically ( f ). MMC simulations show an initial CsCl crystal ( j ) transforming ( k ) into a stable final CuAu-FCC structure with HCP-like stacking faults ( l ). Images show a rendered section through the crystallite, coloured using common neighbour analysis: blue (BCC), red (HCP) and green (FCC). Full size image Further evidence for a diffusionless transformation came from additional NEMC simulations based on the same interaction model used to generate the phase diagram shown in Fig. 3b . In these simulations, spherical crystallites having a CsCl symmetry (with 2,000 particles) were introduced into an otherwise empty simulation box with periodic boundary conditions. The particles were subjected to an interaction matrix for which CuAu-FCC is the lowest free-energy phase [15] ( E AA =1.2 k b T , E AB =5 k b T ). The NEMC simulations were performed using small displacements (<0.001 of the particle diameter), consistent with a Brownian trajectory [26] . Following an initial equilibration phase in which the crystallites equilibrated with a dilute particle ‘vapour’ phase, we found that crystallites reproducibly underwent diffusionless transformations to a CuAu-FCC structure. The transformations typically required about 1–3 million Monte Carlo move attempts per particle before initiation but then proceeded rapidly to completion. Control runs in which the ‘like’ interactions were reduced to zero did not exhibit solid–solid transformations of any kind and the crystallites remained in the CsCl configuration. Crystal structure was analysed using common neighbour analysis within the OVITO software package (www.ovito.org). Briefly, common neighbour analysis first identifies particles that are nearest-neighbours of a given reference particle. The cutoff distance for identifying nearest-neighbours was chosen to be either 446 nm (for identifying CsCl) or 386 nm (for CuAu). A topological graph is then constructed on the basis of the nearest-neighbour particles and used to identify the local crystal structure. Notably, the simulated transformations consistently yielded a higher density of stacking faults ( Fig. 4j-l ) than the experimental case. The precise details of the transformation and its nucleation were complex and will be the subject of a future publication. We have previously shown [15] that stacking faults in CuAu-FCC can have essentially zero energy cost, making their prevalence dependent on kinetic factors, which are presumably not captured properly within the NEMC simulations. Experimentally, the fraction of CsCl crystals that transform is observed to depend monotonically on the DNA-mixing ratio α with up to 76% conversion for the α =0.16 case ( Fig. 3a ). Such incomplete conversion is consistent with slower kinetics for initiating the transformation, and correspondingly fewer stacking faults, which depend on the free energy driving as dictated by α . Last, additional experimental evidence for the diffusionless transformation comes from a statistical analysis of the crystallites’ faceting. In general, crystallites settle to the coverslip because of gravity and come to rest on a crystal facet. As the confocal viewing plane is parallel to the coverslip, we determine the crystal plane of the facet by identifying the plane of a section through the midplane. Crystals grown from solution typically display facets corresponding to their dense planes, as we find for our CsCl and FCC-SS crystals. In contrast, many of the CuAu crystals display unexpected non-dense {110} planes. The conjectured Bain-like tetragonal deformation has the effect of mapping the observed CsCl {110} facets onto the unexpected CuAu {110} facets ( Supplementary Fig. S4 ), as well as replicating the frequency distribution of all the observed facets’ symmetries to within statistical uncertainty (see Supplementary Table S2 ). In conclusion, the major motivation for using DNA handshaking to assemble particles is to utilize its designable matrix of mutual, specific interactions between different particle species to assemble unique nanoparticle and nanocolloid materials. As with atomic materials, however, assembling these new ‘synthetic atoms’ to create clusters, bulk crystals, thin films and heterojunctions will require detailed understanding of how they nucleate, grow, anneal and transform under controlled processing conditions. Our observations reveal that these materials behave like atomic materials [16] in a key manner during thermal processing—by nucleating and growing in one kinetically accessible phase, and then spontaneously transforming into a second phase having a lower free energy. This in turn suggests that many of the thermal and mechanical processes used to control crystal domain size and texture should have analogies in the controlled processing of these new DNA handshaking materials. Moreover, it appears that conventional particle-level simulations with empirical potentials and material science principles should suffice to design and understand the processing behaviour of these materials. Particle preparation Sixty-five bases-long DNA strands, 5′ amine modified, are custom synthesized by IDT DNA. Five hundred milligram of F108 Pluronic (BASF), 100 mg of 4-nitrophenol chloroformate (NCPF), 30 μl of triethylamine (TEA), and 2 ml of dichloromethane (Sigma-Aldrich) are mixed on ice for 2 h. The dissolved F108 is rinsed by adding 15 ml of a mixture of EtOH: HCl (40:1, −20 °C) and after 2 h at −20 °C, is collected by centrifugation and rinsed with a mixture of EtOH: HCl (160:1, −20 °C). Activated F108 is vacuum dried overnight. Fifteen milligram of activated F108 is dissolved in 1 ml of 10 mM citric acid buffer at pH 4. Fifteen microliter of DNA strands (490 μM in water), previously mixed with 1 μl of 1 M carbonate buffer at pH 9, are mixed with 4 μl of F108 solution at room temperature for 2 h. DNA strands are covalently attached to F108 molecules. A final volume of 400 μl per particle type per α at 1% particle volume fraction is targeted. Here, we need 14 samples, 7 α values and two particle types. For this, we mix 105 μl of 490 μM DNA strand ‘ s ’ solution in water with 7 μl of 1 M carbonate buffer and react thoroughly with 28 μl of activated F108 solution. An identical procedure is performed simultaneously for the complementary strands . Finally, each solution is diluted with 2,296 μl of biological water. An A species sample at α =0.06 is obtained by adding 327 μl of strand ‘ s ’ solution with 21 μl of strand solution, forming a final solution of 348 μl. The two populations of strands are mixed thoroughly before grafting. This methodology applies to the remaining samples. A swelling/deswelling technique is used to graft the DNA-labeled copolymers to colloidal particles [18] . Three hundred forty-eight microliter of the DNA-F108 solution described above is mixed with 40 μl of 10% (v/v) of 405 nm solid carboxylate-modified latex (medium acid) particles (Seradyn) and 8 μl of 500 m M Tris buffer pH 8. To fluorescently-label the particles, we add 4 μl of dye–toluene solution at a concentration of 0.02 mg ml −1 for the green Bodipy (4,4-difluoro-5-(2-thienyl)-4-bora-3a,4a-diaza-s-indacene-3-dodecanoic acid) to tag A or 0.024 mg ml −1 for the red Bodipy (4,4-difluoro-1,3,5,7,8-pentamethyl-4-bora-3a,4a-diaza-s-indacene) to tag B; the dyes are obtained from Invitrogen. Toluene is removed by steam stripping the dispersion at 90 °C for 4 min on a hot plate. Finally, samples are washed five times in a 1:10 ratio of 1XTE (pH=8) by centrifugation and re-dispersion to remove excess F108, DNA strands and DNA-grafted-F108. The final sample consists of 400 μl solution of 1% DNA-grafted, fluorescently tagged particles in 1XTE. Fluorescently stained DNA-grafted colloids exhibit similar binding thermodynamics to non-stained particles (identical melting temperatures). Particle crystal formation In a 200-μl PCR tube, 3.5 μl of 23% A spheres, 3.5 μl of 23% B spheres are mixed with 1 μl of a 8XTE, 800 mM NaCl solution so that the final solution contains 8 μl of DNA-grafted colloids at 20% volume fraction at 1XTE, pH 8 and 100 mM NaCl, which are suitable conditions for the DNA strands hybridization. After mixing both particle species together, resulting aggregated samples were melted by brief heating, suspended and mixed while hot, and then cooled slowly at a rate of ~0.3 °C per h while submerged in a 34-l, thermally insulated hot water bath. We estimate that crystal nucleation, growth and transformation occur once the interactions become sufficiently strong, which will occur at different times and temperatures for different α values. Control experiments were performed attempting to crystallize one-component suspensions of just A or B particles at different α values, starting at 20% particle volume fraction. As in α =0.5 samples, crystals formed that structurally resembled the FCC-SS crystals described in the main text. The α =0.21 samples formed a mixture of small FCC crystals and aggregates. Like-interactions for lower α samples were too weak to drive assembly at room temperature and no crystals or aggregates were found. These findings are consistent with our understanding of interactions, crystal nucleation and growth in our system. Confocal imaging To enable confocal visualization, our concentrated crystal samples were diluted with buffer and mounted in microscopy chambers. To reduce photobleaching of the crystal structures during the acquisition, samples are mounted using a SlowFade solution obtained from Invitrogen. Typically, 1 μl of the 8 μl of DNA-grafted colloids at 20% volume fraction is mixed with 20 μl of a buffer made with 100 mM NaCl, 1XTE at pH 8 and 20 μl of SlowFade. A thin ridge of vacuum grease on a glass coverslip is drawn following a square of about 5 mm on each side. 5 μl of colloidal solution is carefully placed within. A clean coverslip is deposited on top of the sample to seal it. Presence of salt in the hybridization buffer is sufficient to immobilize the structures onto the glass via electrostatic interactions. High resolution fluorescent images are acquired using a VTEye confocal (VisiTech) connected to an inverted microscope (Leica DM-IRB equipped with an NA 1.4 × 100 oil immersion objective and an oil condenser). An immersion oil with a refraction index of 1.530 (Type A, Cargille Laboratories) is used. Red Bodipy is excited by a 568-nm laser line while the green Bodipy is excited by a 488-nm laser line. Each image acquisition results from averaging 20 frames to reduce random noise. To accurately register and merge our two-colour images for rendering, we correct for slight optical offsets and distortions introduced by the scan optics of our confocal microscope. To quantify the offset, we use 1 μm carboxylate-modified latex microspheres that are simultaneously stained with the two relevant fluorophores, and thus visible in both channels, immobilized on a microscope slide. The centroids of these colloids serve as fiducial markers. Their differing coordinates in the two colour images, determined by particle tracking routines [27] , are used to translate and dewarp the red channel image into registration with the green, using built-in routines in the Interactive Data Language. Image distortion is <1% near the centre of the field of view, so does not significantly affect the inferred lattice spacing between particles. Subsequently, ImageJ is used to merge, render and adjust the colour contrast of our two-colour micrographs. Phase diagram calculations Phase diagrams were computed by first estimating the amount of compositional disorder present in a superlattice crystal under prescribed growth conditions. The compositional disorder was estimated based on equilibrium ordering isotherms computed previously [15] . These isotherms were used to calculate N AB , the average number of unlike neighbours per particle, for both CuAu and CsCl structures according to the expressions where E anti is the difference between the potential energy well depth of an unlike particle pair and a like particle pair. For a given superlattice structure degree of compositional ordering, free energies were computed using two different methods. The first method was the QHA [21] . In this approach the free energy of a system is determined by calculating vibrational and enthalpic free energy contributions separately. The vibrational free energy is obtained by computing the eigenvalues, w n 2 , of the Hessian matrix for the desired crystal phase, that is, where m is the particle mass, N is the total number of positive eigenvalues, K b is the Boltzmann constant, T is the temperature and λ T is the thermal de Broglie wavelength. The enthalpic contribution is then calculated by where N tot is the total number of particles and N AB and N AA are, respectively, the average number of unlike and like neighbours per particle. The total free energy is then found by summing these two contributions. The second method used for calculating free energy was thermodynamic integration [22] . In this approach, a new potential, U λ , is defined as where U 0 is some reference potential for which the free energy is known (Hookean spring potential), U 1 is the interaction potential experienced by the real system and λ is a scaling parameter. A series of Brownian dynamics simulations were then run at values of λ ranging from 0 to 1 with step sizes of 0.05. For each of these simulations, the average potential energy of the system subject to both the reference potential and the DNA potential was calculated separately. These values are then used to calculate the free-energy difference between the real system and the reference system using the expression How to cite this article : Casey, M.T. et al . Driving diffusionless transformations in colloidal crystals using DNA handshaking. Nat. Commun. 3:1209 doi: 10.1038/ncomms2206 (2012).